Phosphorylation of ARPP19 by protein kinase A prevents meiosis resumption inXenopusoocytes During oogenesis, oocytes are arrested in prophase and resume meiosis by activating the kinase Cdk1 upon hormonal stimulation. In all vertebrates, release from prophase arrest relies on protein kinase A (PKA) downregulation and on the dephosphorylation of a long sought but still unidentified substrate. Here we show that ARPP19 is the PKA substrate whose phosphorylation at serine 109 is necessary and sufficient for maintaining Xenopus oocytes arrested in prophase. By downregulating PKA, progesterone, the meiotic inducer in Xenopus , promotes partial dephosphorylation of ARPP19 that is required for the formation of a threshold level of active Cdk1. Active Cdk1 then initiates the MPF autoamplification loop that occurs independently of both PKA and ARPP19 phosphorylation at serine 109 but requires the Greatwall (Gwl)-dependent phosphorylation of ARPP19 at serine 67. Therefore, ARPP19 stands at a crossroads in the meiotic M-phase control network by integrating differential effects of PKA and Gwl, two kinases essential for meiosis resumption. The well-conserved cAMP-dependent protein kinase A (PKA) is the major mediator of the pleiotropic cellular regulator, cAMP [1] . PKA is composed of two catalytic (C) and two regulatory (R) subunits that keep the enzyme inactive. The binding of cAMP to PKA-R dissociates active PKA-C, which regulates biological processes including memory, differentiation, proliferation and metabolism. While most of its contribution involves the activation of gene transcription, non-genomic effects of PKA have been implicated in M-phase progression by modulating MPF (M-Phase promoting factor) activity, the universal inducer of cell division in eukaryotes [2] , [3] , [4] . Remarkably, high PKA activity is responsible for arresting vertebrate oocytes at the diplotene stage of prophase of the first meiotic division (prophase I) through an unknown post-transcriptional mechanism that ultimately inhibits MPF activation [5] . This arrest lasts over long periods (from months to years depending on species) and allows cell growth by nutrient accumulation and intracellular reorganization that are essential for the success of fertilization and embryogenesis. Hence, the identification of the PKA-phosphorylated protein(s) responsible for arresting oocytes in prophase I is one of the major issues in sexual reproduction. Release from prophase arrest is triggered at the time of ovulation by a hormonal signal, progesterone (Pg) in Xenopus . Oocytes complete the first meiotic division and halt at metaphase of the second meiotic division (MII), awaiting to be fertilized, a feature common to all vertebrate species. This transition from prophase I to MII, called meiotic maturation, depends on the activation of MPF, a complex between the kinase Cdk1 (cyclin-dependent kinase 1) and its regulatory subunit, cyclin B. MPF activation relies on the dephosphorylation of Cdk1 ensured by the activation of the phosphatase Cdc25 (cell division cycle 25) and the concomitant inhibition of the kinase Myt1 (membrane-associated tyrosine-and threonine-specific cdc2-inhibitory kinase). Active MPF then triggers entry into the first meiotic division [6] , which starts with nuclear envelope breakdown, referred to as germinal vesicle breakdown (GVBD) in oocytes. In Xenopus oocytes, Pg inhibits adenylyl cyclase, resulting in a 20% decrease in cAMP level and leading to PKA inhibition within 1 h independently of protein synthesis [7] , [8] , [9] , [10] . The negative action of PKA on meiotic resumption is conserved in all vertebrate species and was discovered in experiments modulating either intracellular cAMP levels or the activity of PKA in oocytes [11] . In mice, the maintenance of high cAMP levels by a pharmacological blockade of phosphodiesterases (PDEs), by the activation of adenylyl cyclases or by adding dibutyryl-cAMP to the external medium prevents oocyte meiotic maturation [5] . Moreover, knockout of the Pde3A gene prevents meiotic resumption [12] . In Xenopus , the injection of PKA-C blocks Pg-induced entry into meiosis I [13] . Conversely, the injection of PKA-R or the heat-stable PKA inhibitor, PKI, induces oocyte maturation in the absence of Pg [13] , [14] , [15] , [16] . This implies that the phosphorylation of one or more PKA substrates is responsible for prophase arrest of vertebrate oocytes. The downregulation of PKA activity induced by Pg is both necessary and sufficient for the dephosphorylation of these critical PKA substrate(s) leading to meiotic resumption. However, the identity of the oocyte PKA substrate(s) is still unknown. PKA has been proposed to directly phosphorylate Cdc25 and inhibit its activation [17] . However, the timing of Cdc25 dephosphorylation, occurring at the time of MPF activation 3–5 h after Pg stimulation, cannot account for the effects and consequences of the rapid inactivation of PKA in these cells. Therefore, the identity of the crucial PKA substrate(s) in oocytes remains an open question. Biochemical steps linking PKA downregulation to MPF activation include the translation of two proteins. One is the kinase Mos, which indirectly activates MAPK (mitogen-activated protein kinase) (the Mos/MAPK pathway) and contributes to Myt1 inhibition and Cdc25 activation [18] , [19] , [20] , [21] , [22] . The second is cyclin B, which associates with free Cdk1 molecules to form new Cdk1 active complexes [23] , [24] . By the coordinated action of cyclin B and Mos, whose synthesis occurs downstream of PKA inhibition [23] , a ‘starter’ amount of active Cdk1 is generated, which then initiates the MPF amplification loop [25] . This autoamplification loop relies on the hyperphosphorylation of Cdc25 and Myt1 by Cdk1 itself but also implicates other kinases such as the Xenopus polo-like kinase (Plx1), the Mos/MAPK pathway and Greatwall (Gwl) [26] , [27] , [28] , [29] , [30] , [31] , [32] , [33] , [34] . The effects of Gwl on M-phase progression are mediated by the phosphorylation at serine 67 (S67) of a close relative to α-endosulfine, the small heat-stable protein ARPP19 (cAMP-regulated phosphoprotein-19) [35] , [36] , [37] , [38] . ARPP19 is in this way converted into a potent inhibitor of PP2A-B55δ, an event necessary for Cdk1 activation in Xenopus oocytes thus launching the MPF autoamplification loop [32] , [36] , [37] , [38] . While the early transduction pathway induced by Pg and leading to the initial activation of Cdk1 depends on PKA downregulation, the MPF autoamplification loop does not. Indeed, transferring cytoplasm from an MII-arrested oocyte, the traditional assay for activating the MPF autoamplification loop [39] , promotes meiotic resumption in prophase oocytes even in the presence of high PKA activity [32] , [40] . This process is ensured by S67-phosphorylated ARPP19 that allows M-phase progression independently of PKA activity [32] . Interestingly, ARPP19 is also a major cytosolic substrate of PKA. This protein is efficiently phosphorylated at serine 107 (S107, equivalent to S109 in Xenopus ARPP19) by PKA in various cell lines and in the striatum, mediating PKA actions in these systems [35] , [41] . Intriguingly, in an attempt to search for the PKA substrate(s) responsible for prophase arrest, a 20 kDa phosphoprotein was partially purified from Xenopus oocytes by virtue of its acid solubility and thermostability but the molecular identity of this protein was not further analysed [42] . Since its biochemical characteristics are astonishingly similar to ARPP19, we reasoned that this PKA substrate could be ARPP19. Here, we demonstrate that ARPP19 is the long sought crucial PKA substrate in oocytes. This protein stands at a crossroads in the meiotic cell cycle control network by integrating PKA and Gwl regulatory signals to control Cdk1 activation and meiosis resumption. Exogenous ARPP19 inhibits Pg-induced maturation In 1986, a 20 kDa substrate of PKA partially purified from Xenopus oocytes was proposed to be responsible for prophase arrest [42] . However, further investigation of this protein was not continued and its molecular identity was not revealed. Using the purification protocol described in Boyer et al ., [42] the heat- and acid-stable fractions obtained from prophase and MII-arrested oocytes were immunoblotted with a specific ARPP19 antibody revealing the presence of this protein in both fractions ( Fig. 1a ). However, in our hands, this fraction purified from prophase oocyte did not modify Pg-induced maturation when injected in oocytes. We incidentally noticed that the phosphorylation of this 20 kDa protein was not preserved during the purification procedure, probably accounting for the absence of effects on meiotic maturation. Nevertheless, we tested the ability of ARPP19 to modulate M-phase entry by injecting various amounts of purified recombinant WT-GST-ARPP in prophase-arrested oocytes. Meiotic maturation was then triggered by addition of Pg (1 μM) and the percentage of GVBD was plotted as a function of time ( Fig. 1b ). The injection of 77.5 ng per oocyte (2 μM final concentration) of WT-GST-ARPP accelerated Pg-induced GVBD ( Fig. 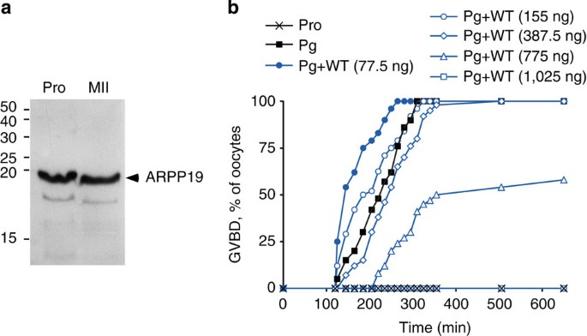Figure 1: Overexpression of ARPP19 in prophase oocytes has a dual effect on meiotic maturation induced by Pg. (a) ARPP19 is present in fractions from prophase (Pro) and MII-arrested (MII) oocytes extracted by trichloroacetic acid precipitation and heat treatment. ARPP19 was immunoblotted using a specific ARPP19 antibody. (b) High amounts of injected WT-GST-ARPP inhibit meiotic maturation. Prophase-arrested oocytes (Pro) were injected with indicated concentrations of WT-GST-ARPP (WT, blue lines). After Pg stimulation, GVBD time course was followed. See alsoSupplementary Table 1. 1b , Supplementary Table 1 ), in agreement with a previous study [32] . However, increasing the amount of injected WT-GST-ARPP led to a dose-dependent inhibition of GVBD ( Fig. 1b , Supplementary Table 1 ). Figure 1: Overexpression of ARPP19 in prophase oocytes has a dual effect on meiotic maturation induced by Pg. ( a ) ARPP19 is present in fractions from prophase (Pro) and MII-arrested (MII) oocytes extracted by trichloroacetic acid precipitation and heat treatment. ARPP19 was immunoblotted using a specific ARPP19 antibody. ( b ) High amounts of injected WT-GST-ARPP inhibit meiotic maturation. Prophase-arrested oocytes (Pro) were injected with indicated concentrations of WT-GST-ARPP (WT, blue lines). After Pg stimulation, GVBD time course was followed. See also Supplementary Table 1 . Full size image ARPP19 is phosphorylated at S109 by PKA in prophase oocyte In mammalian cells, ARPP19 is phosphorylated by PKA at S107, which corresponds to S109 in Xenopus . To investigate the phosphorylation state of ARPP19 at S109 during meiotic resumption, we designed a specific antibody directed against the phosphorylated S109 residue of Xenopus ARPP19 ( Supplementary Fig. 1 ). Prophase-arrested oocytes were collected at the indicated times after Pg addition. Meiotic maturation was assessed by monitoring the phosphorylation of Cdk substrates and MAPK that starts at GVBD ( Fig. 2a ). ARPP19 protein level was stable during meiotic maturation as revealed by an anti-ARPP19 antibody and was phosphorylated at S109 in prophase ( Fig. 2a ). Pg led within 60 min to a partial dephosphorylation of ARPP19 at S109 (mean=49%, s.d.=19, n =4) ( Fig. 2b ). 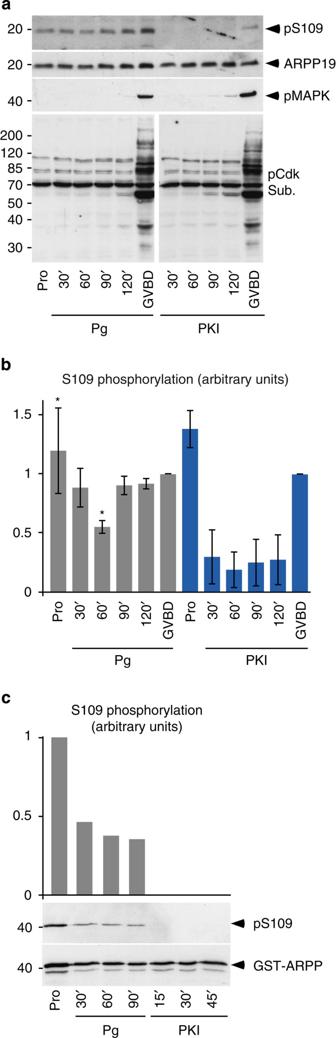Figure 2: ARPP19 is phosphorylated at S109 by PKA in prophase-arrested oocytes and is partially dephosphorylated in response to Pg. (a) ARPP19 phosphorylation at S109 in oocytes. Prophase-arrested oocytes (Pro) were treated either with Pg or injected with PKI then collected at the indicated times. Oocyte lysates were analysed by western blot for S109-phosphorylated ARPP19 (pS109), phosphorylated MAPK, phosphorylated Cdk1 substrates (pCdk Sub.) and total ARPP19. (b) S109 phosphorylation level of ARPP19 was quantified using ImageJ software. The error bars represent means±s.e.m. Asterisks (*) indicate significant difference from prophase oocytes withP<0.05 (Student’st-test,n=4 for Pg-treated oocytes andn=3 for PKI-injected oocytes). (c) Recombinant WT-GST-ARPP is phosphorylated by PKA in prophase oocytes and is dephosphorylated following Pg stimulation. Prophase-arrested oocytes (Pro) were injected with 77.5 ng of WT-GST-ARPP then 15 min later stimulated by Pg or injected with PKI. Oocytes were collected at the indicated times, WT-GST-ARPP was pulled down and isolated fractions were immunoblotted for phosphorylated WT-GST-ARPP19 at S109 (pS109) and total ARPP (GST-ARPP). ARPP19 was then progressively rephosphorylated at S109, reaching or exceeding the prophase level at the time of GVBD ( Fig 2a,b ). Figure 2: ARPP19 is phosphorylated at S109 by PKA in prophase-arrested oocytes and is partially dephosphorylated in response to Pg. ( a ) ARPP19 phosphorylation at S109 in oocytes. Prophase-arrested oocytes (Pro) were treated either with Pg or injected with PKI then collected at the indicated times. Oocyte lysates were analysed by western blot for S109-phosphorylated ARPP19 (pS109), phosphorylated MAPK, phosphorylated Cdk1 substrates (pCdk Sub.) and total ARPP19. ( b ) S109 phosphorylation level of ARPP19 was quantified using ImageJ software. The error bars represent means±s.e.m. Asterisks (*) indicate significant difference from prophase oocytes with P <0.05 (Student’s t -test, n =4 for Pg-treated oocytes and n =3 for PKI-injected oocytes). ( c ) Recombinant WT-GST-ARPP is phosphorylated by PKA in prophase oocytes and is dephosphorylated following Pg stimulation. Prophase-arrested oocytes (Pro) were injected with 77.5 ng of WT-GST-ARPP then 15 min later stimulated by Pg or injected with PKI. Oocytes were collected at the indicated times, WT-GST-ARPP was pulled down and isolated fractions were immunoblotted for phosphorylated WT-GST-ARPP19 at S109 (pS109) and total ARPP (GST-ARPP). Full size image To determine whether PKA could be responsible for ARPP19 phosphorylation at S109 in prophase, oocytes were injected with the specific PKA protein inhibitor, PKI, then collected at the indicated times. As expected, PKI injection triggered GVBD and Cdk1 activation as seen by MAPK and Cdk substrate phosphorylation ( Fig. 2a ). Under this condition, S109 phosphorylation of endogenous ARPP19 was strongly reduced within 30 min following PKI injection and increased again towards the baseline level at the time of GVBD, despite the presence of PKI ( Fig 2a,b ). When oocytes were first injected with PKI then by WT-GST-ARPP 15 min later, the recombinant WT-GST-ARPP was never phosphorylated at S109, except at GVBD time ( Supplementary Fig. 2 ). Therefore, ARPP19 is phosphorylated at S109 by PKA in prophase oocytes, then partially dephosphorylated 1 h following Pg stimulation and is rephosphorylated by a kinase likely distinct from PKA at the time of GVBD. In Xenopus oocytes, the downregulation of PKA induced by Pg occurs independently of protein synthesis [9] . Hence, the dephosphorylation of PKA substrate(s) induced by Pg should be insensitive to protein synthesis inhibition. We therefore incubated prophase oocytes with a protein synthesis inhibitor, cycloheximide 1 h before adding Pg ( Supplementary Fig. 3 ). The partial dephosphorylation of ARPP19 at S109 was still induced by Pg when protein synthesis was inhibited ( Supplementary Fig. 3 ), demonstrating that this event occurs downstream of PKA, independently of protein synthesis. Finally, we ascertained that recombinant WT-GST-ARPP was phosphorylated at S109 by PKA in intact prophase oocytes ( Fig. 2c ). Prophase oocytes were injected with WT-GST-ARPP then either incubated with Pg or injected with PKI. As expected, exogenous ARPP19 was phosphorylated at S109 in prophase oocytes ( Fig. 2c ). Pg induced a significant dephosphorylation of WT-GST-ARPP at S109 within 30 min whereas PKI injection induced full dephosphorylation of WT-GST-ARPP at S109 within 15 min ( Fig. 2c ). Therefore, recombinant WT-GST-ARPP is phosphorylated by PKA in prophase oocytes and is dephosphorylated in response to Pg, mimicking the endogenous ARPP19. S109 phosphorylation prevents Pg-induced meiotic resumption To address the role of ARPP19 dephosphorylation at S109 during meiotic resumption, we generated two recombinant ARPP19 mutants: a phosphomimetic S109D-GST-ARPP and a non-phosphorylatable S109A-GST-ARPP. A third mutant, S67A-GST-ARPP, which cannot be phosphorylated by Gwl at S67 and blocks Pg-induced meiotic maturation [32] , was used as a control. These three mutant proteins were injected in prophase oocytes and their effects on meiosis resumption were monitored ( Fig. 3 ). Injection of WT-GST-ARPP (775 ng per oocyte) delayed Pg-induced GVBD, as already shown in Fig. 1b , whereas the same amount of S109A-GST-ARPP had little effect compared with Pg alone ( Fig. 3a ). Under these conditions, Cdk1 was activated as seen by the phosphorylation of one of its substrates, Cdc27, and the activation of the Mos/MAPK pathway ( Fig. 3b ). In contrast, S109D-GST-ARPP completely abolished Pg-induced GVBD ( Fig. 3a ) as well as Cdk1 activation ( Fig. 3b ). 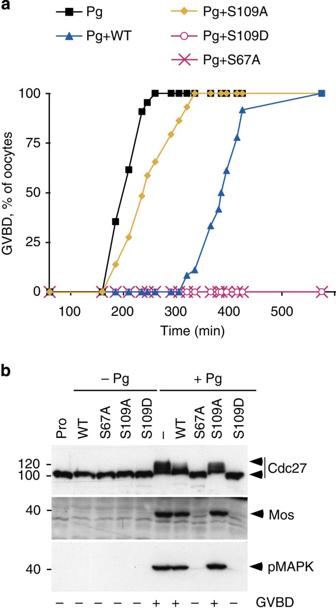Figure 3: S109 phosphorylation of ARPP19 prevents the prophase release of the oocyte in response to Pg. (a) Injection of S109D-GST-ARPP inhibits GVBD induction by Pg. GVBD time course induced by Pg in prophase-arrested oocytes injected with 775 ng of WT-, S67A-, S109A- or S109D-GST-ARPP. (b) S109D-GST-ARPP prevents Cdk1 activation induced by Pg. Oocytes from the experiment described in panel (a) were collected at GVBD and lysates were immunoblotted for Cdc27 phosphorylation, Mos accumulation and phosphorylated MAPK (pMAPK). As expected, meiotic resumption and Cdk1 activation were also prevented by the injection of S67A-GST-ARPP ( Fig 3a,b ). In those oocytes, WT-, S67A- and S109D-GST-ARPP were not phosphorylated at S67 and did not interact with PP2A-B55δ whereas the S109A mutant was phosphorylated at S67 and efficiently interacted with PP2A-B55δ ( Supplementary Fig. 4 ). Therefore, when ARPP19 phosphorylation at S109 is maintained, oocytes remain arrested in prophase despite stimulation by Pg. This suggests that partial dephosphorylation of ARPP19 at S109 is necessary for meiotic M-phase entry and Cdk1 activation in response to Pg. Figure 3: S109 phosphorylation of ARPP19 prevents the prophase release of the oocyte in response to Pg. ( a ) Injection of S109D-GST-ARPP inhibits GVBD induction by Pg. GVBD time course induced by Pg in prophase-arrested oocytes injected with 775 ng of WT-, S67A-, S109A- or S109D-GST-ARPP. ( b ) S109D-GST-ARPP prevents Cdk1 activation induced by Pg. Oocytes from the experiment described in panel ( a ) were collected at GVBD and lysates were immunoblotted for Cdc27 phosphorylation, Mos accumulation and phosphorylated MAPK (pMAPK). Full size image It is known that PKI, like Pg, induces GVBD in a dose-dependent manner [13] , [14] , [15] . This suggests that the dephosphorylation level of the PKA substrate should vary as a function of Pg concentration. Initially, we found that as more WT-GST-ARPP is injected in prophase, more phospho-S109 ARPP19 is generated in these cells due to high PKA activity ( Supplementary Fig. 5 ). Moreover, the efficiency of WT-GST-ARPP in preventing GVBD was increased at lower concentrations of Pg whereas S109D-GST-ARPP inhibited GVBD with the same efficiency at any concentrations of Pg ( Supplementary Fig. 6 ). As expected, S109A-GST-ARPP neither promoted GVBD on its own nor facilitated GVBD in the presence of sub-optimal doses of Pg ( Supplementary Fig. 6 ). Together, these results suggest that meiotic resumption depends on the level of S109 phosphorylation and that this level depends on the Pg concentration in the external media. Increasing Pg concentration should therefore overcome the blockade of maturation induced by the injection of high amounts of WT-GST-ARPP. To address this question, prophase oocytes were injected with either WT- or S109D-GST-ARPP (600 ng per oocyte) then incubated with the usual concentration of Pg (1 μM). For this high amount of WT-GST-ARPP, GVBD was not induced after 16 h ( Fig. 4a ) and Cdk1 was not activated, as shown by Cdk1 phosphorylation at Y15, cyclin B2 electrophoretic migration, as well as MAPK and Gwl phosphorylation ( Fig. 4b ). 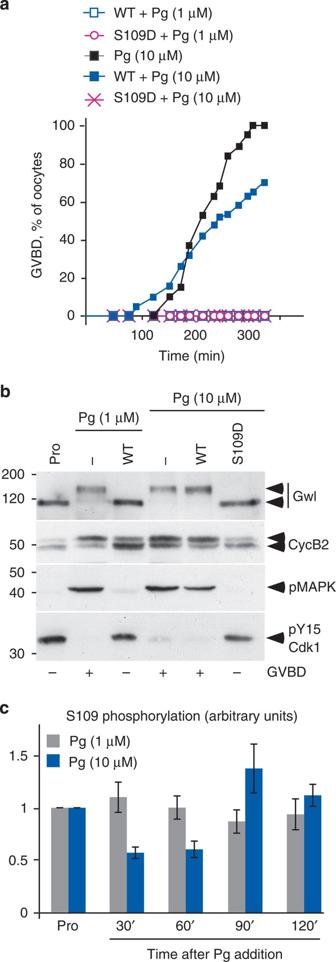Figure 4: The inhibitory effect of injected WT-GST-ARPP on meiotic resumption depends on the concentration of Pg. (a) GVBD time course of WT- or S109D-injected oocytes in response to increased concentrations of Pg. Prophase-arrested oocytes (Pro) were injected with 600 ng of either WT- or S109D-ARPP then stimulated with 1 μM of Pg. 16 h later, no maturation was observed. Injected oocytes were further incubated with 10 μM of Pg in the external media and the GVBD time course was followed. (b) Increasing the concentration of progesterone promotes Cdk1 activation in WT-GST-ARPP injected oocytes. Prophase-arrested oocytes (Pro) or Pg-treated oocytes (Pg) from panel (a) were collected 16 h after 1 μM Pg stimulation or at the time of GVBD in response to 10 μM Pg. Oocytes were analysed by immunoblotting Gwl, cyclin B2 (CycB2) upshift, phosphorylated MAPK (pMAPK) and Cdk1 phosphorylation at Y15 (pY15-Cdk1). (c) The extent of ARPP19 dephosphorylation at S109 depends on Pg concentration. Prophase-arrested oocytes were injected with 600 ng of WT-GST-ARPP then induced to mature either with 1 μM or 10 μM of Pg. Oocytes were collected after Pg addition at the indicated times. The phosphorylation at S109 and the total amount of WT-GST-ARPP were immunoblotted using a specific phospho-S109 and a GST antibody, respectively. S109 phosphorylation level of ARPP19 was further quantified using ImageJ software (n=6). The error bars represent means±s.e.m. After 16 h, Pg concentration was raised to 10 μM for both WT- or S109D-injected oocytes ( Fig 4a,b ). At this elevated concentration, Pg was able to trigger GVBD and Cdk1 activation in oocytes injected with 600 ng of WT-GST-ARPP ( Fig 4a,b ). In contrast, 10 μM Pg was unable to promote meiotic resumption of S109D-GST-ARPP-injected oocytes. We next ascertained the phosphorylation level of WT-GST-ARPP at S109 in response to these two concentrations of Pg ( Fig. 4c ). WT-GST-ARPP was weakly dephosphorylated at S109 in response to 1 μM Pg whereas its dephosphorylation at S109 was increased in response to 10 μM Pg ( Fig. 4c and Supplementary Fig. 7 ). Therefore, the extent of S109 dephosphorylation is regulated by the concentration of Pg and accounts for the negative effect of ARPP19 on meiosis resumption. Figure 4: The inhibitory effect of injected WT-GST-ARPP on meiotic resumption depends on the concentration of Pg. ( a ) GVBD time course of WT- or S109D-injected oocytes in response to increased concentrations of Pg. Prophase-arrested oocytes (Pro) were injected with 600 ng of either WT- or S109D-ARPP then stimulated with 1 μM of Pg. 16 h later, no maturation was observed. Injected oocytes were further incubated with 10 μM of Pg in the external media and the GVBD time course was followed. ( b ) Increasing the concentration of progesterone promotes Cdk1 activation in WT-GST-ARPP injected oocytes. Prophase-arrested oocytes (Pro) or Pg-treated oocytes (Pg) from panel ( a ) were collected 16 h after 1 μM Pg stimulation or at the time of GVBD in response to 10 μM Pg. Oocytes were analysed by immunoblotting Gwl, cyclin B2 (CycB2) upshift, phosphorylated MAPK (pMAPK) and Cdk1 phosphorylation at Y15 (pY15-Cdk1). ( c ) The extent of ARPP19 dephosphorylation at S109 depends on Pg concentration. Prophase-arrested oocytes were injected with 600 ng of WT-GST-ARPP then induced to mature either with 1 μM or 10 μM of Pg. Oocytes were collected after Pg addition at the indicated times. The phosphorylation at S109 and the total amount of WT-GST-ARPP were immunoblotted using a specific phospho-S109 and a GST antibody, respectively. S109 phosphorylation level of ARPP19 was further quantified using ImageJ software ( n =6). The error bars represent means±s.e.m. Full size image Initial Cdk1 activation requires S109 dephosphorylation While PKA downregulation is essential for triggering Cdk1 activation in response to Pg, a high level of PKA activity has no effect on the MPF autoamplification loop [16] , [25] , [32] , [43] . As a key substrate for PKA, ARPP19 dephosphorylation at S109 should therefore be required for Cdk1 activation induced by Pg but not for the MPF autoamplification process. To determine whether ARPP19 dephosphorylation at S109 is involved in the initial activation of Cdk1, prophase oocytes were injected with WT- or S109D-GST-ARPP (300 ng per oocyte) and meiotic maturation was triggered by Pg or by injecting PKI, Mos or a non-degradable form of cyclin B (Δ90). All these proteins lead to the formation of a starter amount of Cdk1 in a PKA-dependent manner, upstream of the autoamplification loop [15] , [16] , [17] , [40] , [44] , [45] . The presence of WT-GST-ARPP did not impair Cdk1 activation in response to Pg, PKI or Δ90-cyclin B injection as seen by Gwl activation, cyclin B2 upshift, MAPK phosphorylation, Cdk1 dephosphorylation at Y15 and Cdk1 substrate phosphorylation ( Fig. 5a ). In contrast, injecting S109D-GST-ARPP prevented Cdk1 activation induced by Pg, PKI or Δ90-cyclin B ( Fig. 5a ). Similarly, the injection of Mos was unable to activate Cdk1 in the presence of the S109D mutant ( Fig. 5b ). Under these conditions, Mos-induced MAPK activation was abolished by the injection of S109D-GST-ARPP in agreement with previous results showing that high PKA activity prevents activation of MAPK by Mos [44] . Our results demonstrate that ARPP19 is the crucial substrate of PKA that needs to be dephosphorylated to generate the threshold level of active Cdk1, which consequently fires the autoamplification process. 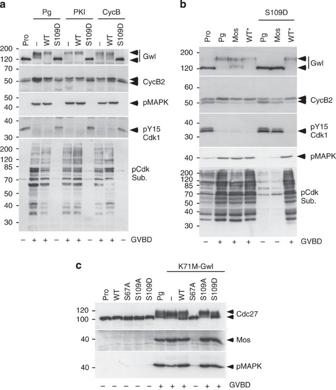Figure 5: S109 phosphorylation of ARPP19 prevents the initial activation of Cdk1 required for meiosis resumption. (a) Injection of S109D-GST-ARPP inhibits Cdk1 activation induced either by PKI or cyclin B. Prophase-arrested oocytes (Pro) were injected with 300 ng of WT- or S109D-GST-ARPP then induced to mature by Pg or by injecting either a non-degradable form of cyclin B (CycB) or PKI. Oocytes were collected at GVBD and Cdk1 activation was followed by immunoblotting Gwl, cyclin B2 (CycB2), MAPK phosphorylation (pMAPK), Cdk1 phosphorylation at Y15 (pY15-Cdk1) and phosphorylated Cdk1 substrates (pCdk Sub). (b) Injection of S109D-GST-ARPP prevents Mos-induced Cdk1 activation but does not inhibit meiotic resumption induced by S67-thiophosphorylated WT-GST-ARPP. Prophase-arrested oocytes (Pro) were injected or not with 300 ng of S109D-GST-ARPP (S109D) then induced to mature by progesterone (Pg) or by injecting either Mos or S67-thiophosphorylated WT-GST-ARPP (WT*). Oocytes were collected at GVBD and immunoblotted for Gwl, cyclin B2 upshift (CycB2), Cdk1 phosphorylation at Y15 (pY15-Cdk1), phosphorylated MAPK (pMAPK) and phosphorylated Cdk1 substrates (pCdk Sub). (c) Injection of S109D-GST-ARPP does not inhibit Cdk1 activation induced by K71M-Gwl. Prophase-arrested oocytes (Pro) were injected with WT-, S67A-, S109A- or S109D-GST-ARPP and meiotic maturation was triggered by the injection of mRNA encoding K71M-Gwl. Oocytes were collected 18 h later and immunoblotted for phosphorylated Cdc27, Mos accumulation and phosphorylated MAPK (pMAPK). Figure 5: S109 phosphorylation of ARPP19 prevents the initial activation of Cdk1 required for meiosis resumption. ( a ) Injection of S109D-GST-ARPP inhibits Cdk1 activation induced either by PKI or cyclin B. Prophase-arrested oocytes (Pro) were injected with 300 ng of WT- or S109D-GST-ARPP then induced to mature by Pg or by injecting either a non-degradable form of cyclin B (CycB) or PKI. Oocytes were collected at GVBD and Cdk1 activation was followed by immunoblotting Gwl, cyclin B2 (CycB2), MAPK phosphorylation (pMAPK), Cdk1 phosphorylation at Y15 (pY15-Cdk1) and phosphorylated Cdk1 substrates (pCdk Sub). ( b ) Injection of S109D-GST-ARPP prevents Mos-induced Cdk1 activation but does not inhibit meiotic resumption induced by S67-thiophosphorylated WT-GST-ARPP. Prophase-arrested oocytes (Pro) were injected or not with 300 ng of S109D-GST-ARPP (S109D) then induced to mature by progesterone (Pg) or by injecting either Mos or S67-thiophosphorylated WT-GST-ARPP (WT*). Oocytes were collected at GVBD and immunoblotted for Gwl, cyclin B2 upshift (CycB2), Cdk1 phosphorylation at Y15 (pY15-Cdk1), phosphorylated MAPK (pMAPK) and phosphorylated Cdk1 substrates (pCdk Sub). ( c ) Injection of S109D-GST-ARPP does not inhibit Cdk1 activation induced by K71M-Gwl. Prophase-arrested oocytes (Pro) were injected with WT-, S67A-, S109A- or S109D-GST-ARPP and meiotic maturation was triggered by the injection of mRNA encoding K71M-Gwl. Oocytes were collected 18 h later and immunoblotted for phosphorylated Cdc27, Mos accumulation and phosphorylated MAPK (pMAPK). Full size image Phospho-S109 ARPP19 does not inhibit MPF autoamplification We next investigated the dependency of the MPF autoamplification loop upon ARPP19 phosphorylation at S109. For this purpose, we used S67-phosphorylated ARPP19 that activates Cdk1 by stimulating directly the MPF autoamplification loop independently of PKA activity [32] . WT-GST-ARPP was thiophosphorylated in vitro by Gwl at S67 (pS67-WT-GST-ARPP) and injected in prophase oocytes. Cdk1 activation was efficiently promoted by pS67-WT-GST-ARPP as previously described [32] and, importantly, still occurred in the presence of the S109D-GST-ARPP ( Fig. 5b ). Meiotic resumption was then induced by injecting oocytes with messenger RNA (mRNA) encoding a constitutive form of Gwl (K71M-Gwl) in the presence of WT-, S109A-, S109D-GST-ARPP or a mutant that cannot be phosphorylated by Gwl, S67A-GST-ARPP ( Fig. 5c ). All these proteins except the S67A mutant were unable to prevent meiotic maturation in response to K71M-Gwl as seen by Cdc27 phosphorylation and the activation of the Mos/MAPK pathway ( Fig. 5c ). We then used classical experimental procedures to directly launch the MPF autoamplification loop, either by injecting okadaic acid (OA) or by transferring the cytoplasm of MII-arrested oocytes (CT) in WT- or S109D-GST-ARPP-injected prophase oocytes ( Fig. 6a ). We also incubated oocytes in the presence of the phosphodiesterase inhibitor, 1-methyl-3-isobutylxanthine (IBMX), known to maintain high cAMP levels and high PKA activity in oocytes [46] . As expected, either IBMX or S109D-GST-ARPP prevented Cdk1 activation and GVBD in response to Pg ( Fig. 6a ). On the contrary, after OA injection or CT, Cdk1 was activated despite the presence of IBMX, confirming the independence of the MPF autoamplification from PKA [47] , [48] , [49] ( Fig. 6a ). In agreement with this result, OA injection and CT were able to activate Cdk1 in the presence of the phosphomimetic S109D-GST-ARPP ( Fig. 6a ). Therefore, the MPF autoamplification loop is independent of PKA activity and, most importantly, functions independently of PKA-phosphorylated ARPP19. 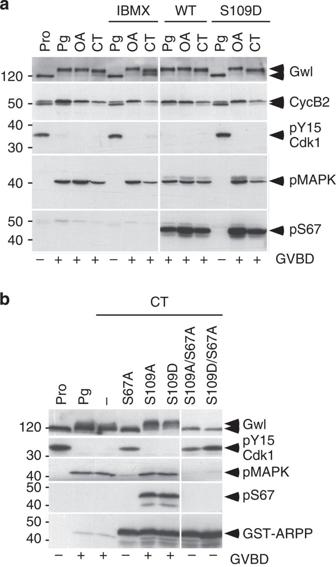Figure 6: The MPF autoamplification loop is independent of ARPP19 phosphorylation at S109. (a) S109D-GST-ARPP does not inhibit Cdk1 activation induced by okadaic acid (OA) injection or cytoplasmic transfer (CT). Prophase-arrested oocytes (Pro) were injected with 400 ng of WT- or S109D-GST-ARPP (S109D) then induced to mature either with Pg, by injecting OA or by transferring cytoplasm from MII-arrested oocytes (CT). Oocytes treated with Pg, injected with OA or CT were previously incubated with IBMX for 1 h. Oocytes were collected at time of GVBD and immunoblotted for Gwl, cyclin B2 upshift (CycB2), Cdk1 phosphorylation at Y15 (pY15-Cdk1), phosphorylated MAPK (pMAPK) and S67-phosphorylated ARPP (pS67). (b) Prophase-arrested oocytes (Pro) were injected with 400 ng of S67A-, S109A-, S109D-, S109A/S67A- or S109D/S67A-GST-ARPP then induced to mature by transferring cytoplasm from MII-arrested oocytes (CT). Some oocytes were induced to mature with Pg as a control. Oocytes were collected at GVBD and immunoblotted for Gwl, Cdk1 phosphorylation at Y15 (pY15-Cdk1), phosphorylated MAPK (pMAPK), S67 phosphorylation of GST-ARPP (pS67) and GST (GST-ARPP). Figure 6: The MPF autoamplification loop is independent of ARPP19 phosphorylation at S109. ( a ) S109D-GST-ARPP does not inhibit Cdk1 activation induced by okadaic acid (OA) injection or cytoplasmic transfer (CT). Prophase-arrested oocytes (Pro) were injected with 400 ng of WT- or S109D-GST-ARPP (S109D) then induced to mature either with Pg, by injecting OA or by transferring cytoplasm from MII-arrested oocytes (CT). Oocytes treated with Pg, injected with OA or CT were previously incubated with IBMX for 1 h. Oocytes were collected at time of GVBD and immunoblotted for Gwl, cyclin B2 upshift (CycB2), Cdk1 phosphorylation at Y15 (pY15-Cdk1), phosphorylated MAPK (pMAPK) and S67-phosphorylated ARPP (pS67). ( b ) Prophase-arrested oocytes (Pro) were injected with 400 ng of S67A-, S109A-, S109D-, S109A/S67A- or S109D/S67A-GST-ARPP then induced to mature by transferring cytoplasm from MII-arrested oocytes (CT). Some oocytes were induced to mature with Pg as a control. Oocytes were collected at GVBD and immunoblotted for Gwl, Cdk1 phosphorylation at Y15 (pY15-Cdk1), phosphorylated MAPK (pMAPK), S67 phosphorylation of GST-ARPP (pS67) and GST (GST-ARPP). Full size image Since ARPP19 is rephosphorylated at S109 at GVBD, we next ascertained that the MPF autoamplification process was strictly dependent on S67 phosphorylation of ARPP19 and not on its phosphorylation at S109. For this purpose, we generated two double mutants of ARPP19 that cannot be phosphorylated at S67 by Gwl (S67A) and containing point mutations at S109: the non-phosphorylatable S109A and the phosphomimetic S109D. When these two double mutants, S109A/S67A or S109D/S67A, were injected in prophase-arrested oocytes, they completely abolished GVBD induction and Cdk1 activation in response to Pg ( Supplementary Fig. 8 ). The MPF autoamplification loop was then activated by CT in prophase oocytes previously injected with either S109A/S67A- or S109D/S67A-GST-ARPP (400 ng per oocyte) ( Fig. 6b ). As controls, prophase oocytes were also injected with the single mutants S109A-, S109D- or S67A-GST-ARPP. None of the S109 single mutants was able to block Cdk1 activation induced by CT. Gwl was activated, MAPK was phosphorylated, Cdk1 was dephosphorylated at Y15 and GST-ARPP was phosphorylated at S67 ( Fig. 6b ). In contrast, CT was no longer able to promote Cdk1 activation when oocytes were injected either with S67A-, S109A/S67A- or S109D/S67A-GST-ARPP ( Fig. 6b ). Therefore, the MPF autoamplification loop relies entirely on S67 phosphorylation of ARPP19 regardless of the phosphorylation status of S109. By western blot, we further determined that S109D-GST-ARPP was in vivo phosphorylated at S67 following the activation of the MPF autoamplification loop with OA or CT ( Fig 6a,b ). Therefore, the phosphorylation at S109 of ARPP19 does not prevent its phosphorylation at S67 by Gwl nor its MPF inducing activity. Altogether, these results demonstrate that ARPP19 phosphorylation at S109 controls the formation of a starter amount of active Cdk1 but the MPF autoamplification loop, subsequently launched by this threshold level of active Cdk1, is independent of this phosphorylation. Once activated, Gwl phosphorylates ARPP19 at S67 and from this point S109 phosphorylation loses its biological inhibitory effects on Cdk1 activation. In all vertebrate oocytes, the phosphorylation of an unknown protein by PKA arrests the first meiotic division in prophase for long periods. The dephosphorylation of this crucial actor is a pre-requisite for the resumption of meiosis at the time of ovulation. In amphibian oocytes, Pg releases prophase arrest by inducing a transient decrease in adenylyl cyclase activity, cAMP levels and PKA activity within 1 h [7] , [8] , [9] , [10] . The molecular connection between the substrate of PKA and Cdk1 activation remains elusive. Cdc25 and Wee1 are phosphorylated by PKA in oocytes [17] , [50] , [51] . Interestingly, not only these two direct regulators of Cdk1 but also other contributors to Cdk1 activation including the Mos/MAPK pathway or the module Gwl-ARPP19-PP2A are unable to promote meiotic maturation in a high PKA context, except ARPP19 phosphorylated at S67 by Gwl [15] , [16] , [17] , [20] , [21] , [28] , [29] , [30] , [31] , [32] , [33] , [40] , [44] , [45] . This indicates that PKA inhibits oocyte maturation at two periods: at the early steps of the signalling pathway within the first hour following hormonal stimulation, and at the level of the molecular components required for Cdk1 activation 3 to 4 h later. The identity of the PKA substrate regulating the early step of meiosis resumption remains an open question in vertebrates. Recently, the substrate of the Gwl kinase, the small protein ARPP19, was shown to play a central role in M-phase progression through PP2A inhibition [36] , [37] , [38] . In Xenopus , ARPP19 phosphorylated at S67 by Gwl promotes Cdk1 activation by launching the MPF autoamplification loop independently of PKA activity [32] . Interestingly, ARPP19 stands for ‘cAMP-regulated phosphoprotein’ and is phosphorylated by PKA in many mammalian cells [35] . Intriguingly, in 1986, a phosphoprotein of 20 kDa was partially purified from Xenopus oocytes by virtue of its acid solubility and thermostability [42] . This protein was described as an in vivo substrate of PKA, was dephosphorylated 1 to 2 h following Pg treatment, and was thought to block meiotic maturation when injected under its phosphorylated form [42] . Given the similarities between the biochemical characteristics of this unidentified protein and ARPP19, we hypothesized that ARPP19 could be the key component maintaining the oocyte arrested in prophase. We show here that ARPP19 phosphorylation at S109 by PKA is essential and sufficient for maintaining oocyte prophase arrest, as the S109D phosphomimetic mutant blocks Pg- and PKI-induced prophase release. This result was further validated using exogenous WT-GST-ARPP, which blocks meiotic resumption in a dose-dependent manner. Increasing the amount of WT-GST-ARPP increases the level of ARPP19 phosphorylated at S109, mimicking PKA inhibitory effects on meiotic entry. The inhibitory effect of high amounts of WT-GST-ARPP can be bypassed by increasing the concentration of Pg that stimulates dose-dependently the extent of ARPP19 dephosphorylation at S109. Altogether, our results strongly argue that the inhibitory effect of injected ARPP19 depends on the level of phosphorylated WT-GST-ARPP at S109 left in the oocyte following Pg stimulation. Since the extent of ARPP19 dephosphorylation at S109 depends on Pg concentrations, this illustrates for the first time the proportionality between the concentration of steroids, the downregulation of PKA, the dephosphorylation of its substrate and the ability of the oocyte to mature. Further investigation will be therefore necessary to understand how a minor part of dephosphorylated ARPP19 (49%) can carry out this function despite the presence of the S109 inhibitory phosphoform of the protein. Moreover, a major issue in the future will be to identify the phosphatase responsible for ARPP19 dephosphorylation at S109. In Xenopus oocyte, GVBD is promoted by Cdk1 activation that obeys a two-step mechanism [52] . During the first step, the downregulation of PKA and the synthesis of new proteins are required to generate a threshold level of active Cdk1 [25] . This starter amount of active Cdk1 then initiates the MPF autoamplification loop that occurs independently of protein synthesis and PKA downregulation as ascertained by cytoplasm transfer experiments [16] , [43] . It is therefore expected from a substrate of PKA that its phosphorylated form would abolish Cdk1 activation whereas its dephosphorylation would allow the formation of the threshold level of active Cdk1. Indeed, ARPP19 dephosphorylation at S109 is necessary for the activation of Cdk1 in response to Pg and its phosphomimetic form, S109D-GST-ARPP, fully blocks inducers of maturation like cyclin B, PKI or Mos. On the other hand, the injection of OA, S67-thiophosphorylated ARPP19, K71M-Gwl or cytoplasm transfer can directly trigger the MPF autoamplification loop without the need of a threshold level of active Cdk1. Interestingly, these treatments are able to bypass the S109D-ARPP19 blockade of meiotic maturation. In conclusion, ARPP19 has to be dephosphorylated at S109 to generate the threshold level of active Cdk1. Once the MPF autoamplification loop is initiated, ARPP19 phosphorylation at S109 loses its biological inhibitory effect. In addition, ARPP19 is unexpectedly rephosphorylated at S109 when oocytes enter the first meiotic division, an event no longer apparently fulfilled by PKA since it takes place in the presence of PKI. An important question is therefore to understand why S109-phosphorylated ARPP19 no longer has an inhibitory effect when the MPF autoamplification loop is fired. In a previous study, we demonstrated that the phosphorylation of ARPP19 at S67 by Gwl at GVBD switches ARPP19 into an effective inducer of Cdk1 through PP2A-B55δ inhibition and this phosphorylation renders the MPF autoamplification independent of PKA activity [32] . Since the phosphorylation of S109 does not prevent the phosphorylation of ARPP19 at S67 once the MPF autoamplification loop is fired, it will be important to investigate the functional interplay between S67 phosphorylation and S109 phosphorylation of ARPP19 within the early transduction pathway induced by Pg. Another major issue will be to decipher the molecular mechanism connecting the dephosphorylated form of ARPP19 at S109 and the activation of Cdk1. We previously showed that S67 phosphorylation of ARPP19 depends on Cdk1 activation in Xenopus oocytes [32] . Since S109D-GST-ARPP prevents the initial activation of Cdk1 induced by Pg and has no effect on meiosis resumption when oocytes are injected with S67-phosphorylated WT-GST-ARPP, this strongly suggests that the S109D mutant may not act by preventing S67-phosphorylated ARPP19 to interact with and inhibit PP2A. However, S109 phosphorylation of ARPP19 could slow down its phosphorylation by Gwl at S67, an event that has to be tightly controlled since it promotes meiosis resumption independently of PKA activity [32] . In yeast, it was also shown that ARPP19 phosphorylation by PKA and Gwl are involved in the control of protein synthesis when cells exit from their quiescence state [53] , [54] . Protein synthesis is a major step required for Cdk1 activation in Xenopus and it would be worthwhile to determine whether this process could be regulated by ARPP19 dephosphorylation at S109 in our model system. We therefore propose that S109-phosphorylated ARPP19 locks the oocyte in prophase whereas the S67-phosphorylated form is necessary for M-phase entry ( Fig. 7 ). Upon Pg stimulation, PKA is inhibited leading to partial dephosphorylation of ARPP19 at S109. This could allow ARPP19 to either interact weakly with PP2A-B55δ thus inhibiting its activity or to be efficiently phosphorylated by Gwl. Concomitantly, PKA and/or ARPP19 could control protein synthesis of either Mos or cyclin B that are required for increasing Cdk1 activity and subsequently for Gwl activation. ARPP19 is thereafter fully phosphorylated at S67, resulting in a strong inhibition of PP2A allowing the autoamplification loop of MPF to take place through the Cdc25/Myt1 balance. From this moment, all processes become independent of protein synthesis and PKA activity and drive the cell into M-phase in an irreversible manner. Therefore, ARPP19 is at a crossroad in the M-phase control network, integrating PKA signalling to halt cell cycle in G2 with Gwl to induce M-phase by linking Cdk1 activation to PP2A-B55δ. 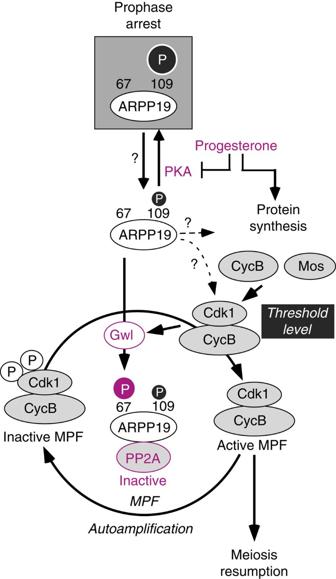Figure 7: Schematic representation of the regulation of meiotic resumption by ARPP19 inXenopusoocytes. During oogenesis, the phosphorylation of ARPP19 by PKA at S109 is responsible for arresting oocytes in prophase I. In response to Pg, PKA activity is downregulated and, as a consequence, ARPP19 is partly dephosphorylated at S109. ARPP19 dephosphorylation at S109 is necessary to generate the threshold level of active Cdk1 by either facilitating ARPP19 phosphorylation at S67 or by controlling protein synthesis. Once a starter amount of active Cdk1 is formed, it initiates the MPF autoamplification loop. Gwl is activated under the control of Cdk1 and fully phosphorylates ARPP19 at S67, launching the MPF autoamplification independently of PKA activity and, thus, of ARPP19 phosphorylation at S109. At that time, meiotic M-phase entry becomes irreversible. Figure 7: Schematic representation of the regulation of meiotic resumption by ARPP19 in Xenopus oocytes. During oogenesis, the phosphorylation of ARPP19 by PKA at S109 is responsible for arresting oocytes in prophase I. In response to Pg, PKA activity is downregulated and, as a consequence, ARPP19 is partly dephosphorylated at S109. ARPP19 dephosphorylation at S109 is necessary to generate the threshold level of active Cdk1 by either facilitating ARPP19 phosphorylation at S67 or by controlling protein synthesis. Once a starter amount of active Cdk1 is formed, it initiates the MPF autoamplification loop. Gwl is activated under the control of Cdk1 and fully phosphorylates ARPP19 at S67, launching the MPF autoamplification independently of PKA activity and, thus, of ARPP19 phosphorylation at S109. At that time, meiotic M-phase entry becomes irreversible. Full size image In mammalian cultured cells, cAMP level fluctuates being high in interphase, and low in M-phase [55] and the elevation of cAMP blocks somatic cells in G2 whereas its reduction or the injection of PKI triggers mitosis [4] , [56] , [57] . Thus, PKA seems likely to play an important role in keeping Cdk1 inactive during G2 in the normal mitotic cell cycle. Investigating whether this regulation involves ARPP19 in these systems will be essential. The study of this key physiological process should provide important contributions to knowledge of the hormonal regulation of reproduction, with potential clinical relevance in human fertility and tumorigenesis. Materials Xenopus laevis adult females (Xenopus Express, France) were bred and maintained under laboratory conditions (Animal Facility Agreement: #B75-05-13, all experiments were performed with the approval of the Charles Darwin n° 5 ethics committee). Reagents, unless otherwise specified, were from Sigma. Preparation and handling of Xenopus oocytes Fully grown Xenopus prophase oocytes were obtained as described [20] . The usual microinjected volume was 50 nl per oocyte. Progesterone (Pg), cycloheximide and 1-methyl-3-isobutylxanthine (IBMX) were used in the external medium at the respective concentrations of 2 μM, 355 μM and 1 mM. Okadaic acid (OA) was injected at the final concentration of 10 −5 M. Oocytes were referred to as GVBD when the first pigment rearrangement was detected at the animal pole. Cytoplasm (CT) transfer experiments were performed by aspirating the cytoplasm of MII-arrested oocytes and injecting prophase-arrested oocytes [39] . In all experiments using recombinant ARPP19 proteins, prophase oocytes were injected 18 h before inducing meiotic resumption. However, it is important to note that the amount of injected WT-GST-ARPP inhibiting meiotic maturation varies from one female to another ( Supplementary Table 1 ). Therefore, pilot experiments were performed for each female: in these experiments, prophase oocytes were injected with various amounts of WT-GST-ARPP then treated with Pg 1 h later and meiotic maturation was checked after 18 h. Noteworthy, 300 ng of S109D-GST-ARPP totally abolished Pg-induced maturation regardless of the female Xenopus used. Oocytes were homogenized at 4 °C in 10 volumes of extraction buffer (EB: 80 mM beta-glycerophosphate pH 7.3, 20 mM EGTA, 15 mM MgCl 2 ), centrifuged at 15,000 g for 10 min at 4 °C and lysates used for further analysis. ARPP19 purification by trichloroacetic acid precipitation and heat treatment Prophase- or MII-arrested oocytes were purified as described in ref. 42 . Briefly, oocytes were homogenized in 50 mM Tris, pH 7.4, 75 mM KCl, 50 mM NaF, 10 mM Na 2 HPO 4 , 10 mM ATP, 10 mM EDTA, 0.1 mM PMSF, 10 μM orthovanadate and 5 mM phenylphosphate and centrifuged at 10,000 r.p.m. for 20 min. Proteins from supernatants were further purified by 1% then 15% trichloroacetic acid precipitation at 4 °C for 3 h and centrifuged at 12,000 r.p.m. for 30 min. The pellet was then resuspended in 0.5 M Tris, pH 7.6 and boiled for 10 min at 95 °C. After a last centrifugation step, proteins were dialyzed overnight against 5 mM Tris, pH 7 and concentrated by lyophilization. Antibodies and Western Blot An equivalent of 0.5 oocytes was loaded on 12% SDS polyacrylamide gels [58] and immunoblotted as described [21] . To visualize endogenous ARPP19, the equivalent of 1.5 oocytes was loaded on 15.5% Tris-Tricine gels [59] . The following antibodies were used: phosphorylated MAP kinase, pMAPK (1/1,000, Cell Signaling 9106); cyclin B2 (1/1,000, Abcam ab18250); Mos (1/1,000, Santa Cruz Biotechnology Sc-86); Cdc27 (1/500, BD Transduction Laboratory 610454); Y15-phosphorylated Cdk1, pY15-Cdk1 (1/1,000, Cell Signaling 9111); phosphorylated-Cdk substrates, pCdk Sub. (1/1,000, Cell Signaling 2324) and HRP-conjugated antibody against GST (1/10,000, Sigma A-7340). Specific phospho-S67-ARPP19 (1/500), Gwl, ARPP19, PP2A-C subunit and B55δ antibodies were described in refs 32 , 35 . Specific anti-phospho-pS109 antibody directed against ARPP19 was raised by immunizing rabbits with the following peptide: CQDLPQRKPpSLVASK and then affinity-purified on columns containing the immobilized peptides (Covalab) ( Supplementary Fig. 1 ). Appropriate horseradish peroxidase-labelled secondary antibodies (Jackson Immunoresearch) were revealed by chemiluminescence (Pierce). Full scans of all western blots are supplied in Supplementary Fig. 9 . Quantification of S109 phosphorylation ARPP19 phosphorylation at S109 was quantified using ImageJ software. For each female, the signal corresponding to S109 phosphorylation was normalized to total ARPP19. In Fig. 2b , each experiment was then standardized using the S109-phosphorylated signal obtained at GVBD time in either Pg-treated oocytes or PKI-injected oocytes. In Fig. 4c , since 600 ng of WT-GST-ARPP inhibits GVBD induction in response to 1 μM Pg, we normalized our experiments using the S109-phosphorylated signal obtained from prophase oocytes. Cloning of Xenopus Gwl and GST-ARPP Xenopus wild-type Gwl and point mutant K71M-Gwl, wild-type ARPP19 (WT-GST-ARPP) and S67A-GST-ARPP were cloned according to ref. 32 . GST-ARPP cDNA containing point mutations (S109A, S109D, S109A/S67A and S109D/S67A) were generated using the Quick Change site mutagenesis kit (Stratagene) and were verified by DNA sequencing. mRNA encoding K71M-Gwl were produced using the AmpliCap-Max T3 kit (Epicentre). Expression and purification of recombinant proteins Recombinant GST-ARPP proteins, PKI, non-degradable sea urchin Δ90-cyclin B and MBP-Mos proteins were produced in Escherichia coli by autoinduction [60] and purified as described [23] , [32] , [61] . GST-ARPP and MBP-Mos were purified from bacteria lysed by sonification in 50 mM Tris–HCl, pH 7.3, 0.1 M NaCl, 1 mM EDTA, 1 mM EGTA, 5 mM benzamidine, 1 mg ml −1 lysozyme in the presence of detergents (0.5% Triton, 0.5% Igepal). After a brief centrifugation step, supernatants were loaded onto an equilibrated glutathione–agarose column (for GST-ARPP) (Promega) or Maltose Binding Resin (for MBP-Mos) (NEB), washed and eluted either with 10 mM glutathione or 10 mM maltose in 20 mM Tris–HCl, pH 9, 0.5 M NaCl, 0.1 mM EDTA, 0.1 mM EGTA, 1 mM DTT. The purified proteins were concentrated against polyethylene glycol, dialyzed overnight against PBS (phosphate-buffered saline pH 7.4, 13.7 mM NaCl, 2.7 mM KCl, 4.3 mM KH 2 PO 4 , 1.4 mM Na 2 HPO 4 ) and stored at −80 °C. Bacteria expressing the heat-stable inhibitor protein PKI were lysed in 20 mM Tris, pH 8, 1 mM EDTA and 10% sucrose, sonicated and centrifuged at 10,000 r.p.m. for 15 min at 4 °C. Supernatant was then placed in a boiling water bath and held at 95 °C for 5 min. Denatured proteins were removed by centrifugation and the crude heat-treated extract was adjusted to pH 5.0 with acetic acid. After incubation for 30 min at room temperature, precipitated proteins were removed by centrifugation and the supernatant was dialyzed overnight against 10 mM Tris, pH 8, 1 mM EDTA and 50 mM NaCl. Bacteria expressing sea urchin Δ90-cyclin B were lysed in Buffer A (10 mM Tris, pH 8, 50 mM NaCl, 1 mM EDTA, 5 mM DTT and 0.05% Igepal), sonicated and centrifuged at 12,000 r.p.m. for 15 min at 4 °C. The pellet was then resuspended in Buffer A supplemented with 8 M urea and 30 mM β-mercaptoethanol then dialized overnight against 50 mM Tris-HCl, pH 8, 5 mM MgCl 2 , 100 mM KCl and 30 m M β-mercaptoethanol. The concentrations of all the purified recombinant proteins were measured using the Bradford assay [62] . In vitro thiophosphorylation of WT-GST-ARPP Recombinant WT-GST-ARPP protein was thiophosphorylated in vitro by Gwl (at S67) or PKA (at S109) according to the protocol described in ref. 32 . Active Gwl kinase was obtained by injecting prophase oocytes with mRNA encoding Histidine-tagged Xenopus Gwl. The kinase was then recovered on nickel beads from matured oocyte lysates. Histidine-tagged recombinant PKA (a gift from Susan Taylor, Addgene plasmid #14921) was bacterially expressed by autoinduction [60] and recovered from bacterial lysates on Nickel beads (Qiagen). WT-GST-ARPP (500 μg) was incubated with Gwl or PKA bound to Nickel beads for 90 min at 30 °C in kinase buffer (20 mM Hepes pH 7.4, 2 mM β-mercaptoethanol) in the presence of 1 mM γS-ATP. Supernatants containing S67- or S109-thiophosphorylated GST-ARPP were then recovered after centrifugation and dialyzed against PBS. GST pull down Fifty microlitres of oocyte lysates were incubated for 1 h at 4 °C with 30 μl of GST magnetic beads (Promega). GST beads were recovered, washed in EB and resuspended in an equal volume of loading buffer for western blot analysis. How to cite this article: Dupré, A. et al. Phosphorylation of ARPP19 by protein kinase A prevents meiosis resumption in Xenopus oocytes. Nat. Commun. 5:3318 doi: 10.1038/ncomms4318 (2014).